Phonon hydrodynamics in two-dimensional materials The conduction of heat in two dimensions displays a wealth of fascinating phenomena of key relevance to the scientific understanding and technological applications of graphene and related materials. Here, we use density-functional perturbation theory and an exact, variational solution of the Boltzmann transport equation to study fully from first-principles phonon transport and heat conductivity in graphene, boron nitride, molybdenum disulphide and the functionalized derivatives graphane and fluorographene. In all these materials, and at variance with typical three-dimensional solids, normal processes keep dominating over Umklapp scattering well-above cryogenic conditions, extending to room temperature and more. As a result, novel regimes emerge, with Poiseuille and Ziman hydrodynamics, hitherto typically confined to ultra-low temperatures, characterizing transport at ordinary conditions. Most remarkably, several of these two-dimensional materials admit wave-like heat diffusion, with second sound present at room temperature and above in graphene, boron nitride and graphane. The thermal conductivity of materials is a key property that is attracting much interest both for its role and relevance to thermoelectric waste heat recovery, and for the scientific questions and technological opportunities that are arising in the field of low-dimensional materials (see, for example, refs 1 , 2 for a review). When dimensionality is reduced or the relevant sizes reach microscopic scales (from tens of nanometers to tens of microns), the knowledge developed in the past on conventional bulk crystals becomes insufficient, and novel properties emerge. The prototypical two-dimensional (2D) material, graphene, has the highest known thermal conductivity (even if there is to-date no complete consensus on its actual value [1] ), and unexpected phenomena have been observed experimentally, with, for example, a size dependence in the thermal conductivity for samples reaching the micron scale [3] . This is consistent with the theoretical prediction that heat carriers in graphene can propagate for distances up to the millimetre scale [4] . The origin of such behaviour is under active investigation and much debated, with arguments centring around dimensionality effects [3] , [5] , [6] and the reduction of the scattering phase space [7] . It has been noted that for graphene and boron nitride [4] , [7] , [8] , [9] it is essential to consider the exact solution of the Boltzmann transport equation (BTE) when studying thermal conductivity, and that the widely used single-mode relaxation time approximation (SMA; where individual phonons thermalize independently, without collisions repopulating them) fails in describing correctly thermal transport. This failure arises because the simultaneous interaction of all phonon populations is crucial, and such collective behaviour [4] , [10] can lead to the emergence of composite excitations as the leading heat carriers. Such collective behaviour is driven by the dominance of normal (that is, heat-flux conserving) phonon scattering events, which allow the phonon gas to conserve to a large extent its momentum before other resistive scattering mechanisms can dissipate it away. A phonon gas in such state is said to be in the hydrodynamic regime, because of the similarity with the case of an ideal gas where particles scatter without dissipating momentum. Phonons in the hydrodynamic regime can, under specific conditions, form packets that alter the typical diffusive behaviour of heat and make it propagate as a damped wave, giving origin to the phenomenon of second sound, where a localized heating perturbation generates two sound wavefronts when probed at a certain distance [11] , [12] . This phenomenon has not been extensively studied, as to-date it was possible to observe it only in few materials at cryogenic temperatures (10 K or less): solid helium [13] , sodium fluoride [11] , [14] , bismuth [12] , strontium titanate [15] , [16] (theoretically it is also been hypothesized for diamond [17] ). In this work, we study the lattice thermal conductivity of graphene, graphane, boron nitride, fluorographene and molybdenum disulphide by solving the linearized BTE using a variational approach devised by some of us [18] , [19] that is particularly robust in converging to the exact solution of the BTE under all possible conditions (iterative solutions have limited domains of convergence [20] , [21] , [22] and this is particularly challenging in 2D materials [4] , [7] , because of the collective nature of the excitations). In addition, all calculations are parameter free, as scattering rates and lifetimes for phonon–phonon interactions and for isotopic elastic scattering are computed using phonon frequencies and phonon–phonon interactions from density-functional pertubation theory [23] , [24] , [25] , [26] , [27] , [28] , in a reciprocal-space formulation able to deal with any arbitrary wavevector [29] . Isotopic concentrations of the five materials use the natural abundances (see the Methods section for details). Remarkably, we show that all five materials considered fall into the hydrodynamic regime even at room temperature or above it, and we highlight the persistence of second sound in graphene, graphane and boron nitride at temperatures well-above cryogenic. In graphene at room temperature, second sound propagates over distances of the order of 1 μm, hinting at the possibility of devising thermal devices based on coherent propagation [30] . Last, we also provide validation for the Callaway model of thermal conductivity, developed for heat transport at very low temperatures, and shown here to be valid for these 2D materials up to room temperature and above. Boltzmann transport equation The thermal conductivity k is the quantity, which relates the heat flux Q with a gradient of temperature ∇ T , so that Q =− k ∇ T ; for simplicity, the thermal conductivity, which in general is a tensor, is written as a scalar property, as we are considering only the in-plane conductivity, that is, isotropic. To express k as a function of microscopic quantities, one introduces the out-of-equilibrium phonon distribution n v ( ν = q , s labels collectively the Brillouin zone wavevectors and phonon branches). For small perturbations, n v is linearized around the Bose–Einstein thermal equilibrium distribution so that , and all deviations from equilibrium are expressed by the set of functions F v . Using the microscopic expression of the heat flux [31] , [32] , k can be expressed in terms of microscopic quantities as , where is the energy of the phonon ν , υ ν is the projection of the phonon group velocity on the direction parallel to ∇ T and NV is the volume of the crystal. Thus, k depends on harmonic quantities , which can be computed routinely and inexpensively even from first-principles [23] , [24] , and the challenge is to find the F v deviations from equilibrium. To obtain n v , we solve the linearized BTE [18] where the scattering operator is represented by a matrix of scattering rates acting on the phonon populations n v . We focus here mostly on intrinsic processes and isotopic disorder, so the scattering matrix is built using three-phonon processes and isotopic elastic rates as detailed in refs 19 , 26 ; extrinsic sources of scattering (typically, finite sizes) are discussed in connection with the Poiseuille thermal conductivity regime. For simplicity, the BTE is often solved in the SMA, which relies on the assumption that heat-current is dissipated every time a phonon undergoes a scattering event [18] . Therefore, the phonon distribution relaxes towards thermal equilibrium at a rate which is given by the phonon lifetime τ v , the average time between phonon scattering events at equilibrium. The scattering operator is thus approximated as and the SMA thermal conductivity depends directly on the individual phonon lifetimes: . The comparison between the SMA thermal conductivity as a function of temperature and the exact solution of the BTE is reported in Fig. 1a for all five materials considered here, and the qualitative failure of the SMA at all temperatures becomes immediately apparent. This failure has already been highlighted, for example, for the case of graphene and boron nitride, using either first-principles scattering rates for graphene [4] , [7] or empirical potentials [8] , [9] . As expected, we find that such failure occurs also in graphane and molybdenum disulphide, and, by a smaller amount, in fluorographene, making it common in 2D materials. Interestingly, errors affect also qualitative predictions: for example, the SMA solution predicts graphane to have a conductivity larger than graphene at room temperature. 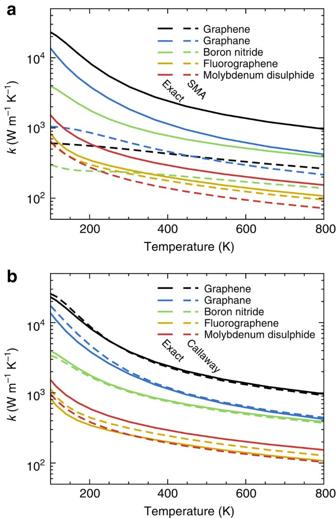Figure 1: Thermal conductivity as a function of temperature. Ab-initioestimates of the thermal conductivitykas a function of temperature for infinite suspended sheets, at natural isotopic abundances. Two approximations are tested against the exact solution of the first-principles phonon Boltzmann transport equation: (a, top panel) the single-mode relaxation time approximation (SMA); (b, bottom panel) Callaway’s model. Figure 1: Thermal conductivity as a function of temperature. Ab-initio estimates of the thermal conductivity k as a function of temperature for infinite suspended sheets, at natural isotopic abundances. Two approximations are tested against the exact solution of the first-principles phonon Boltzmann transport equation: ( a , top panel) the single-mode relaxation time approximation (SMA); ( b , bottom panel) Callaway’s model. Full size image Poiseuille and Ziman hydrodynamics To make further progress, it is very instructive to inspect the scattering rates for the different processes involved, that is, three-phonon processes (divided into normal ( ) and Umklapp ( ) events) and isotopic scattering ( ). For processes, total momentum is conserved and all three phonon wavevectors belong to the first Brillouin Zone, whereas in processes momentum is not conserved, and the sum of the three wavevectors corresponds to a non-zero reciprocal lattice vector. Such distinction is key for heat transport, as it has been long known [18] that processes do not actively dissipate heat-current, as a consequence of energy and momentum conservation, and processes act as the source of intrinsic dissipation. We show in Fig. 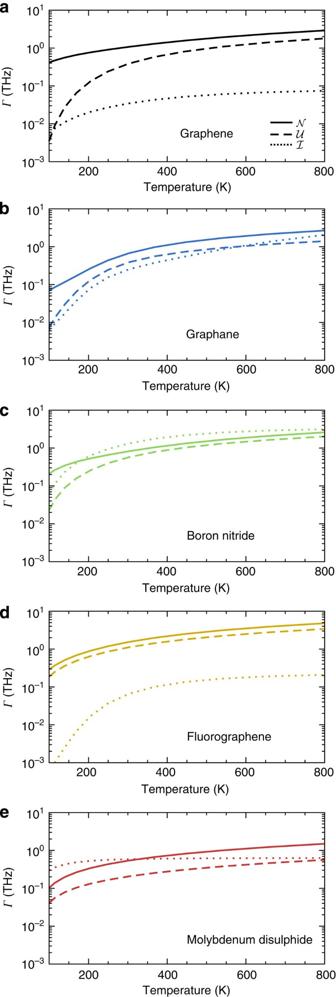Figure 2: Average phonon linewidths. Average linewidths of normal (), Umklapp () and isotopic () scattering processes in infinite suspended sheets of graphene (a), graphane (b), boron nitride (c), fluorographene (d) and molybdenum disulphide (e);processes are calculated at natural isotopic abundances.scattering in all these two-dimensionalmaterials is clearly dominant. 2 the average linewidths for all these processes, defined as Figure 2: Average phonon linewidths. Average linewidths of normal ( ), Umklapp ( ) and isotopic ( ) scattering processes in infinite suspended sheets of graphene ( a ), graphane ( b ), boron nitride ( c ), fluorographene ( d ) and molybdenum disulphide ( e ); processes are calculated at natural isotopic abundances. scattering in all these two-dimensionalmaterials is clearly dominant. Full size image where i labels either , or processes and is the specific heat of the phonon mode ν (this weight is the same appearing in the second-sound velocity shown later). Conventionally, it is expected that events become dominant only at very low temperatures, when processes freeze out [18] , and even then only provided that rates or other extrinsic sources of scattering are negligible. Quite surprisingly, it is seen here that not only processes are very relevant, as argued in refs 8 , 29 , but also that they represent the dominant scattering mechanisms in these 2D materials at any temperature (with the exception of natural-abundance molybdenum disulphide and boron nitride, where is comparable to because of the large isotopic disorder of molybdenum and boron). The predominance of normal scattering processes identifies the regime(s) under which the phonon gas is defined to be in the hydrodynamic conditions mentioned above. We nevertheless underscore that, even if the momentum-conserving nature of processes prevents them from dissipating heat-current, they still affect the total thermal conductivity by altering the out-of-equilibrium phonon distribution. Last, we highlight that the failure of the SMA in these conditions is a rather conceptual one, as it is the assumption that heat flux is dissipated at every scattering event that becomes invalid. Instead, given that most processes are normal, heat flux is just being shuttled between phonon modes. To compare these 2D materials with conventional solids, we summarize in Table 1 the different regimes of phonon transport according to the nomenclature of Guyer [33] . In the ballistic regime, the dominanant scattering events are extrinsic ( ), and are typically due to the finite size of the sample (line defects, surfaces, grain boundaries); in the Poiseuille regime, normal ( ) processes dominate, and the heat flux is dissipated by events (this is the first hydrodynamic regime where the gas of phonons is ‘normal’ but it feels the ‘walls’ of the container). In the Ziman regime, events still dominate, but the heat flux is now dissipated by resistive scattering (either Umklapp ( ) or isotopic ( ))—in this regime, the ‘walls’ have become irrelevant for the normal gas. Finally, in the kinetic regime intrinsic resistive processes (again, typically or ) have the highest linewidth, the sample size is much larger than all typical mean free paths and events have become negligible. Table 1 Classification of thermal transport regimes. Full size table It becomes instructive then to compare graphene, taken as reference, with a typical three-dimensional solid, like silicon or germanium. We show in Fig. 3 the thermal conductivity of graphene both in the case in which we have an infinite sample ( k ∞ ) or a finite ribbon (here of width L =100 μm, k L ), with an extrinsic scattering rate given by (ref. 22 ), considering this also in the ballistic limit obtained by removing all the internal sources of scattering , and , but preserving the extrinsic scattering . The comparison of with the exact thermal conductivity k L in a ribbon of width L shows that the ballistic regime is not a good approximation to k L . In fact, the introduction of scattering events, that is, hydrodynamic conditions, enhances the thermal conductivity well above the ballistic limit. As the thermal conductivity grows with temperature, graphene is in the Poiseuille regime, where events facilitate the heat flux, and extrinsic sources of scattering dissipate it (the term Poiseuille comes from an analogy [33] between the flow of phonons in a material with the flow of a fluid in a pipe). The thermal conductivity though does not grow indefinitely with temperature, because of the limit imposed by the intrinsic thermal conductivity of an infinite sheet k ∞ . Thus, there is a thermal conductivity peak, and for higher temperatures, the heat flux is mostly dissipated by intrinsic sources ( ). As the processes have the largest linewidth at any temperature, the regime at temperatures higher than the peak is still hydrodynamic, but it shifts to Ziman, where the intrinsic resistive processes set the typical length scales, and the boundaries become irrelevant. Last, if the intrinsic events had the largest linewidth, the thermal conductivity would be in the kinetic regime: this is the regime of conventional materials at ordinary temperatures, but it is not ever reached in these 2D cases. 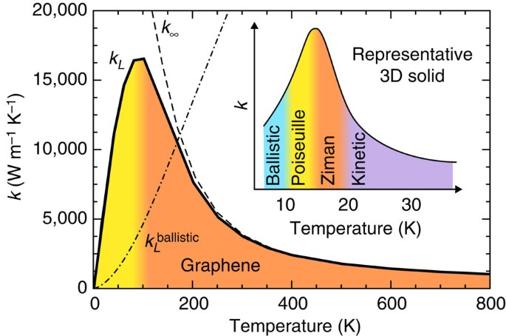Figure 3: Thermal transport regimes in two- and three-dimensional (3D) materials. Thermal conductivity of a graphene ribbon of widthL=100 μm (kL, solid line) together with its ballistic limit (see text;, dashed), and of an infinite graphene sheet (k∞, dashed line). Inset: thermal conductivity regimes in a standard 3D solid (for example, silicon or germanium), where peak conductivity is obtained at cryogenic temperatures and the hydrodynamic conditions, if present, are confined around those temperatures. Figure 3: Thermal transport regimes in two- and three-dimensional (3D) materials. Thermal conductivity of a graphene ribbon of width L =100 μm ( k L , solid line) together with its ballistic limit (see text; , dashed), and of an infinite graphene sheet ( k ∞ , dashed line). Inset: thermal conductivity regimes in a standard 3D solid (for example, silicon or germanium), where peak conductivity is obtained at cryogenic temperatures and the hydrodynamic conditions, if present, are confined around those temperatures. Full size image In conclusion, the two major differences between these 2D materials and a conventional solid are (i) in the temperature scales involved (the non-kinetic regimes in a conventional solid are all condensed in narrow energy window around cryogenic conditions, and hydrodynamic regimes may not be present at all), and (ii) in the fact that even at the highest temperatures normal processes remain dominant, restricting conductivities to just the hydrodynamic regimes of Poiseuille and Ziman. Callaway’s model Callaway’s model is an approximation to the scattering matrix that was originally developed in order to describe the thermal conductivity of germanium at very low temperatures (20 K or so) [34] . It had previously been shown by Klemens [35] that the most probable boson distribution in a system where momentum is conserved is given by the drifting distribution , where V is a Lagrange multiplier enforcing momentum conservation. Therefore, processes will tend to relax the phonon population n v towards . Instead, resistive processes tend to relax the phonon populations towards local thermal equilibrium (that is, the Bose–Einstein distribution ), just as described by the SMA. Therefore, Callaway approximated the scattering operator as where the Matthiessen rule (that is, arithmetic sum of the scattering rates for independent events) is used As scattering rates are very large, an out-of-equilibrium distribution will mostly decay first into the drifting distribution, and from this state it will relax towards static equilibrium. The results for the thermal conductivity in Callaway’s approximation are shown in Fig. 1b , and compared again against the results of the exact solution of the BTE (more details on the expression of Callaway’s thermal conductivity can be found in the Supplementary Note 1 and Supplementary Fig. 1 ). It can be seen that the model broadly reproduces the exact solutions, even if, for example, in fluorographene it overestimates the exact results, or in molybdenum disulphide underestimates them. So, even more than providing simple but fairly accurate estimates of the phonon distribution without the need of solving the BTE, the value of the model is in the clear physical insight it offers on the microscopic nature of heat transport, allowing us to conclude not only that the dominant presence of processes at all temperatures characterizes heat transport in these materials, but also that the distribution function can be broadly described as a drifting distribution according to the prescriptions of Callaway and Klemens [34] , [35] . Second sound Materials in hydrodynamic regimes can host second sound [11] , [12] , [13] , [14] , [15] , [16] , and is thus interesting to discuss its existence or characteristics in two dimensions. We define second sound, following ref. 36 , as the propagation of heat in the form of a damped wave. In a conventional material, one expects only diffusive propagation; it is the ‘second’ heat-wave transport that gives the name to this phenomenon. In principle, more than one microscopic mechanism could lead to the formation of second sound [36] ; the common requirement is that a mechanism exists, which is causing a slow decay of the heat flux. This can indeed happen in case of a large presence of events. As mentioned before, the conservation of momentum drives n v towards , and once this drifting distribution has accumulated, heat propagates as a wave that is eventually damped on longer timescales by the resistive processes that relax the phonons to the equilibrium Bose–Einstein distribution, and determine diffusive heat transport at longer lengths. To observe second sound, the out-of-equilibrium distribution needs to be in the form and well described by the drifting distribution. We have already shown in the previous section that its introduction in the scattering operator provides a good estimate of the thermal conductivity. To see whether the out-of-equilibrium distribution closely resembles the drifting one, we first expand the drifting distribution in a Taylor series, so that it is simply proportional to the projection of the wavevector parallel to the temperature gradient (see Supplementary Note 2 ). Then, we define the drifting component as: which is equal to one if the out-of-equilibrium distribution is equal to the drifting distribution. We plot this quantity for all materials considered in Fig. 4 (as a percentage), and we observe that more than 40% of the phonon distribution of graphene at room temperature is determined by the drifting distribution, and that this ratio grows at lower temperatures; this ratio is slightly smaller in all other materials, falling below 30% for fluorographene and 10% molybdenum disulphide. Therefore, in graphene, graphane and boron nitride, a large fraction of the heat flux is carried by the drifting distribution (which is a good approximation of n v for the study of the heat flux propagation), whereas in fluorographene and molybdenum disulphide, the drifting distribution is a worse descriptor of the out-of-equilibrium distribution, as also hinted by the reduced effectiveness of the Callaway model. 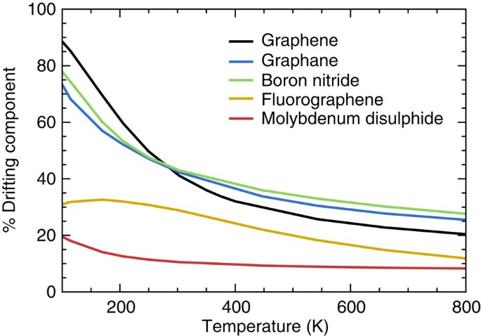Figure 4: Second-sound phonon component. Projection of the out-of-equilibrium phonon distribution onto the drifting distribution (percentage values). Figure 4: Second-sound phonon component. Projection of the out-of-equilibrium phonon distribution onto the drifting distribution (percentage values). Full size image When the drifting distribution is a good approximation to the out-of-equilibrium distribution, the material will display second sound. The second-sound heat wave is characterized by a velocity v ss and a relaxation time τ ss that define a second-sound length λ ss = v ss τ ss , that is, the characteristic distance that the heat wave propagates before decaying. It is possible to show (details are reported in the Supplementary Note 3 ) that, approximating the out-of-equilibrium distribution with the drifting distribution and using the Callaway approximation for the scattering operator, the BTE can be rewritten as a wave-like equation for the temperature profile, characterized by the following quantities: The second-sound relaxation times—reported in the Supplementary Fig. 2 —indicate that the energy flux dissipation decays on average on a time scale of the order of hundred picoseconds at room temperature for the three materials of higher conductivity. The second-sound velocities depend only on harmonic properties, and can be easily computed—they are reported in the Supplementary Fig. 3 as a function of temperature, and compared with the average velocity of acoustic phonons. We find that the different v ss typically lay in between the larger average velocities of the longitudinal and tranverse acoustic branches, and the much lower average velocity of the out-of-plane acoustic mode. The propagation lengths λ ss = τ ss v ss for the second-sound wave for graphene and graphane reach the micron scale, even at room temperature, whereas boron nitride is characterized by second-sound lengths of a fraction of a micron (the values of λ ss for molybdenum disulphide and fluorographene are shown in Fig. 5 for completeness, even if those materials do not host second sound). At lower temperatures, where processes tend to freeze and only are present, damping of the second sound becomes less effective and the heat wave propagates over longer distances. 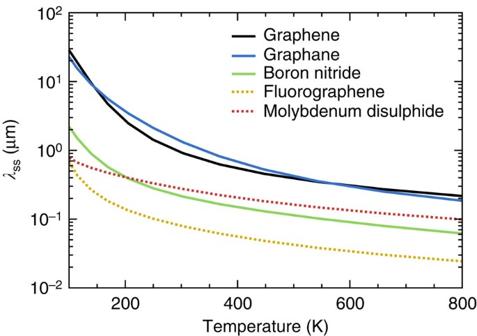Figure 5: Second-sound scattering lengths. Characteristic propagation length of second sound, describing the wave-like propagation of heat. Dotted lines are used for the materials where second sound has a low probability of being observed. We note that for graphene and graphane at room temperature the typical decay length of second sound is of the order of microns. Figure 5: Second-sound scattering lengths. Characteristic propagation length of second sound, describing the wave-like propagation of heat. Dotted lines are used for the materials where second sound has a low probability of being observed. We note that for graphene and graphane at room temperature the typical decay length of second sound is of the order of microns. Full size image As mentioned, the presence of second sound has been verified experimentally in the past [11] , [12] , [13] , [14] , [15] in 3D materials at cryogenic temperatures, and it is conveniently studied as the response of a material to a temperature pulse. One should then be able to observe at a distance standard pulses due to the diffusive propagation by the longitudinal, tranverse and out-of-plane acoustic modes; in addition, the second-sound signature will appear as a further peak due to the formation of the drifting distribution. One should also always consider the size of the experimental setup, as this will affect phonons, which travel ballistically, that is, without scattering between the heat source and the detector, and that would diminish the component of heat travelling in the other modes. Their effect on second sound should be negligible as long as the distance between pump and probe is larger than λ ss . Finally, let us note that the estimate of λ ss is obtained here as a statistical average, and thus we cannot exclude the existence of tails of the second-sound mode propagating at much longer distances. We have investigated heat transport in some key 2D materials—graphene, boron nitride, molybdenum disulphide and the functionalized derivatives graphane and fluorographene. We have found that momentum-conserving normal processes are the dominant scattering mechanisms at all temperatures, requiring an exact solution of the linearized BTE for qualitative and quantitative accuracy, and confirming that graphene provides the highest thermal conductivity among all materials considered. Heat transport in all cases falls into the conditions of Poiseuille and Ziman hydrodynamics (below and above the conductivity peak, respectively), never reaching the ‘ordinary’ conditions of diffusive transport even at very high temperatures. The Callaway model, developed originally for the study of heat transport in conventional three-dimensional solids in the hydrodynamic regimes that could arise at cryogenic temperatures, provides a broadly accurate description of heat transport in two dimensions at all temperatures. Moreover, its microscopic picture of two relaxation time scales, where the out-of-equilibrium distribution accumulates first into a momentum-conserving drifting distribution before relaxing into the final Bose–Einstein equilibrium, provides both microscopic insight and understanding. Graphene, graphane and boron nitride all display second sound, that is, a component in heat transport that behaves as a damped wave and is not described by diffusive propagation, with length scales that reach 1 μm for graphene at room temperature. First-principles simulations Second- and third-order force constants have been calculated using density-functional perturbation theory [23] , [27] , [28] , [37] as implemented in the Quantum ESPRESSO distribution [38] , using the local-density approximation, norm-conserving pseudopotentials from the PSlibrary [39] and a plane-wave cutoff of 90 Ry. The electronic-structure calculations for graphene (G), boron nitride (BN), fluorographene (CF) and graphane (CH) use a Gamma-centred Monkhorst-Pack Brillouin zone sampling of 24 × 24 × 1 k-points, and 16 × 16 × 1 k-points for MoS 2 . All systems are simulated in a supercell geometry, relaxing the in-plane lattice parameter a to equilibrium, and with interlayer distances of 7 Å for all materials except MoS 2 , where it is taken to be 18 Å. For graphene, that is a semimetal, we use a Methfessel-Paxton cold smearing of 0.02 Ry. For all materials, but not for MoS 2 , the harmonic and anharmonic force constants have been computed on meshes of 16 × 16 × 1 and 4 × 4 × 1 q-points in the Brillouin zone, respectively, whereas for MoS 2 they have been computed on 16 × 16 × 1 and 6 × 6 × 1, respectively. Thermal conductivity simulations The BTE is solved using the variational method of ref. 19 , finding well-converged results for a mesh of 128 × 128 × 1 q-points and a Gaussian broadening of 10 cm −1 , except for the case of MoS 2 , where a mesh of 140 × 140 × 1 q-points and a broadening of 1 cm −1 has been used. The isotopic concentrations are chosen to be the natural ones [40] : hydrogen of 99.9885% 1 H, 0.0115% 2 H; carbon of 98.93% 12 C, 1.07% 14 C; boron of 19.9% 10 B, 80.1% 11 B, nitrogen of 99.632% 14 N, 0.368% 15 N; fluorine of 100% 19 F; sulphur of 94.93% 32 S, 0.76 33 S, 4.29 34 S, 0.02% 36 S; molybdenum of 14.84% 92 Mo, 9.25% 94 Mo, 15.92% 95 Mo, 16.68% 96 Mo, 9.55% 97 Mo, 24.13% 98 Mo, 9.63% 100 Mo. The numerical results presented in the text are normalized by the volume of the unit cell of the crystal; the thickness in the perpendicular direction is chosen as the experimental one of the corresponding 3D material, using c/a ratios of 1.367 for graphene and graphane, 1.317 for boron nitride, 1.206 for fluorographene and 1.945 for MoS 2 . All calculations have been managed using the AiiDA materials’ informatics platform [41] . How to cite this article: Cepellotti, A. et al . Phonon hydrodynamics in two-dimensional materials. Nat. Commun , 6:6400 doi: 10.1038/ncomms7400 (2015).